Activation pathway of Src kinase reveals intermediate states as targets for drug design Unregulated activation of Src kinases leads to aberrant signalling, uncontrolled growth and differentiation of cancerous cells. Reaching a complete mechanistic understanding of large-scale conformational transformations underlying the activation of kinases could greatly help in the development of therapeutic drugs for the treatment of these pathologies. In principle, the nature of conformational transition could be modelled in silico via atomistic molecular dynamics simulations, although this is very challenging because of the long activation timescales. Here we employ a computational paradigm that couples transition pathway techniques and Markov state model-based massively distributed simulations for mapping the conformational landscape of c-src tyrosine kinase. The computations provide the thermodynamics and kinetics of kinase activation for the first time, and help identify key structural intermediates. Furthermore, the presence of a novel allosteric site in an intermediate state of c-src that could be potentially used for drug design is predicted. Protein kinases are a family of enzymes that catalyse the transfer of the γ-phosphate group from ATP to the hydroxyl group of specific serine, threonine or tyrosine residues. Their ability to alternate between catalytically active (upregulated) and inactive (downregulated) states in response to specific signals provides a central switching mechanism in cellular transduction pathways, such as in those regulating cellular growth, proliferation and differentiation [1] . Deregulation of kinases can lead to uncontrolled cell proliferation and malignant transformation as observed in numerous cancers [1] , which makes them an important target for therapeutic intervention [2] , [3] . Selective inhibition of kinases using small molecule inhibitors is gaining importance as an effective therapeutic regimen for treatment of a wide range of cancers with the successful approval of imatinib (Gleevec) for treating chronic myeloid leukaemia [4] , [5] . However, despite these encouraging results, this remains very difficult for a number of reasons. Most of the small molecule inhibitors target the ATP-binding pocket in the active/inactive state of the kinase, which is highly conserved owing to the functional similarity between kinases, and therefore provides limited selectivity. Furthermore, targeted protein kinases develop resistance owing to the point mutations in the important structural regions such as the drug-binding site [6] , [7] , [8] , [9] . One of the strategies to overcome molecular resistance and selectivity issues involves targeting kinases by allosteric inhibitors that bind outside the ATP-binding pocket and affect kinase activity by eliciting long-range conformational transformations. While this represents a very promising avenue, the design of allosteric inhibitor is challenging because it not only requires identification of novel allosteric binding sites but also a detailed dynamical picture of allosteric network of residues involved in long-range coupling and activation. Therefore, mechanistic and structural insights into the molecular aspects of kinase conformational change are desired for rational design of selective and robust kinase inhibitors [6] , [9] . The c-src kinase from the Src family of cytoplasmic tyrosine kinases presents an ideal system for mechanistic investigations not only because of its medical and historical relevance [10] but also because of the availability of extensive experimental data related to this kinase including several crystal structures of both inactive and active states [11] . The key structural differences between active and inactive states are the changes in the orientation and conformation of the C-helix in the amino-terminal lobe and the unfolding of the activation loop (A-loop) in the carboxy-terminal lobe ( Fig. 1 ). In the inactive state, the A-loop with unphosphorylated Tyr416 is closed and folded to occlude substrate entry into the active site. In the active state, an outward movement of the A-loop opening up the active site to substrate binding is accompanied by an inward rotation of the C-helix recruiting the residues needed to form a catalytically competent active site. The function of the catalytic domain of c-src is to phosphorylate the tyrosine side chain in a downstream substrate protein, which can also include the Tyr416 in the A-loop from another kinase. It is the process of transphosphorylation of Tyr416 in the A-loop via a bimolecular encounter with another active Src kinase that ‘locks’ the domain in its catalytically active state. To become accessible as a substrate, the A-loop of an inactive kinase must transiently adopt conformations that expose Tyr416 to the solvent. These large-scale conformational changes in the structural elements of kinases are also accompanied by subtle changes in the positions and interactions of specific residues. The active and inactive crystal structures of c-src tyrosine kinase show switching of hydrogen bonding partners of Glu310 from Arg409 to Lys295 (Ozkirimli et al. [12] , [13] ), and the alignment of residues comprising R-spine [14] on activation ( Fig. 1 ). These crystal structures reveal differences between inactive and active conformations but fail to provide insights into the activation mechanism, presence of key intermediates along the activation pathway, the ensemble of pathways connecting the two end states and the timescales of activation/deactivation [5] . It is critical to understand the molecular underpinnings of the kinase activation process to relate these static structures to the kinase function and to provide levers for controlling the activation of aberrant kinase signalling pathways [2] , [3] , [9] . 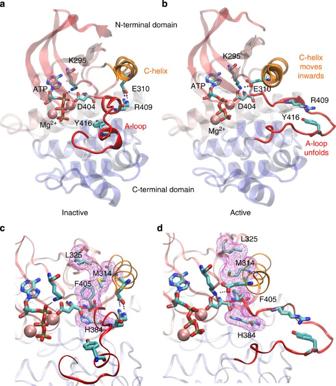Figure 1: Conformational changes associated with the c-src activation. The (a) inactive and (b) active crystal structures show structural changes in the activation loop (A-loop; red) and C-helix (orange), switching of the electrostatic network formed between Lys295, Glu310, Arg409 and Tyr416, and alignment of residues L325, M314, F405 and H384 (shown in licorice and surface representation) to form a hydrophobic regulatory spine (R-spine) in active state (d) as compared with the inactive state conformation (c). R-spine forms a continuous hydrophobic region linking the two lobes of the catalytic domain and it is critical for the catalytic activity of the kinase. Figure 1: Conformational changes associated with the c-src activation. The ( a ) inactive and ( b ) active crystal structures show structural changes in the activation loop (A-loop; red) and C-helix (orange), switching of the electrostatic network formed between Lys295, Glu310, Arg409 and Tyr416, and alignment of residues L325, M314, F405 and H384 (shown in licorice and surface representation) to form a hydrophobic regulatory spine (R-spine) in active state ( d ) as compared with the inactive state conformation ( c ). R-spine forms a continuous hydrophobic region linking the two lobes of the catalytic domain and it is critical for the catalytic activity of the kinase. Full size image Atomistic molecular dynamics (MD) simulations have been used to study conformational transitions in proteins such as the flipping of ‘DFG’ motif [15] , [16] in kinases, calculation of the binding free energy of inhibitors [15] , elucidating activation pathways [17] , [18] , [19] . However, owing to the large system size and long timescales associated with kinase conformational dynamics, most of these studies employ simplifications such as coarse-grain representations of enzymes, ‘enhanced sampling’ techniques, studying mutants with fast conformational transition kinetics [20] , [21] , [22] , [23] , [24] , [25] , [26] , [27] and so on. While simulations have been successful at identifying metastable states of proteins, estimates of the kinetics of conformational transitions have remained elusive because of the challenges outlined above. In the present study, we employ a computational framework that couples transition pathway generation techniques, massively distributed MD simulations (550 μs) on Folding@home [28] , Markov state models (MSMs) and novel adaptive sampling algorithms for mapping the conformational landscape of c-src tyrosine kinase. To sample the conformational landscape more efficiently, we start a large number of relatively short simulations from configurations along an optimal pathway connecting the active (pdb id:1Y57 (Cowan-Jacob et al. [29] )) and inactive (pdb id:2SRC [30] ) states determined using the string method with swarm-of-trajectories. A theoretical framework based on MSM in which conformational dynamics is modelled as transitions between kinetically metastable states is then used to investigate the slow kinetics (~100 μs) of conformational transitions of kinases by using statistical methods to combine a very large number of short trajectories (~20 ns) into a single model [31] , [32] . The MSM analysis of c-src conformational dynamics reveals the presence of key intermediates along the ensemble of c-src activation pathways and for the first time, timescales associated with activation and deactivation processes. The results presented in this study would not only considerably increase our knowledge of the structures of possible intermediate conformations sampled during the kinase activation but also provide an extensive database of c-src conformations for design of future novel kinase inhibitors. Simulations reveal multiple intermediate states of c-src Simulations of c-src catalytic domain are performed in this study. The regulatory SH2 and SH3 domains, which are involved in the autoinhibited inactive state, are not included in the simulations performed in this study to mimic the disassembled upregulated form of the enzyme complex [17] , [30] , [33] . ATP molecule is bound in the nucleotide-binding pocket in the study because of the high likelihood of ATP binding at its physiological concentration of 2–8 mM (Frankel et al. [34] ). The transphosphorylation of Tyr416 locks the kinase domain in the catalytically active state. Tyr416 is phosphorylated owing to encounter with another kinase only when it is exposed to the solvent in an open active-like state as compared with the inactive state of c-src kinase in which it is buried inside the protein surface. In all our simulations, Tyr416 is in an unphosphorylated state. Therefore, the activation transitions observed in this study represent transition between inactive state and an open ‘active-like’ conformation that exposes Tyr416 transiently to another kinase [18] . The starting structures were taken from a minimum free energy pathway (MFEP) connecting the active and inactive state of c-src kinase generated using the string method with swarms-of-trajectories [24] . Analysis of the raw trajectories and MSMs built from the simulation data reveal a detailed conformational landscape of the transitions between active and inactive states of c-src kinase including the kinetics of the dynamical processes occurring on the landscape. The overall strategy that consists of combining the information from multiple trajectories through the use of MSM bears some similarities to that used by Yang et. al. [18] , although the massive configurational sampling involved in the present computations far exceeds any previous study by several orders of magnitude. Analysis of the conformational landscape based on order parameters reveals key intermediates between inactive and active states but fails to provide detailed sequence of events leading to activation, probability of transitions between them, elucidating parallel activation paths and so on. MSMs provide a natural framework for simplified analysis of large simulation data sets by discarding dynamics faster than a certain timescale called lag time [35] instead of projecting the data along a chosen set of order parameters. The Markov state-building process involves separation of the conformational landscape into states with high structural similarity. The transitions between states and the population of each state are obtained by recording the states visited along individual trajectories. A maximum likelihood estimate of the state population and transition probability between states is then obtained, which provides the best model for the kinetics possible, given the data at hand [36] . To ascertain the robustness of the MSM analysis, MSMs with 1,000, 2,000, 3,000, 4,000, 5,000 and 10,000 microstates were built from the simulation data. The implied timescale of the 2,000 state model were converged indicating that the model is Markovian in nature ( Supplementary Fig. 1 ). Therefore, the 2,000 microstate model was chosen for further analysis. Two-dimensional conformational landscape of the c-src tyrosine kinase with respect to several order parameter pairs are shown in Fig. 2 and Supplementary Fig. 2 . Two intermediate states (I 1 and I 2 ) are found along the pathway linking the inactive and active states of c-src kinase. In the intermediate state I 1 ( Fig. 3c ), the A-loop is unfolded but the electrostatic network involving Lys295, Glu310 and Arg409 is in its inactive configuration. In the intermediate state I 2 ( Fig. 3d ), the Glu310-Arg409 hydrogen bond is broken but C-helix has not rotated and moved inwards to facilitate the formation of Lys295-Glu310 hydrogen bond. 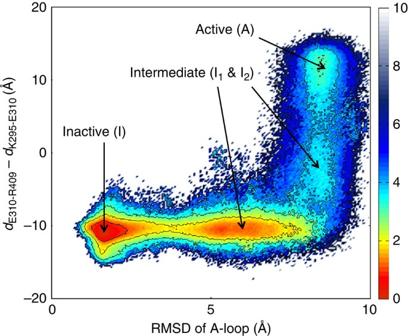Figure 2: Conformational landscape of c-src tyrosine kinase. The conformational landscape generated using r.m.s.d. of A-loop residues (404–424) and difference of the distance between Glu310-Arg409 and Lys295-Glu310 residue pairs as the order parameters reveals multiple intermediates along the activation pathway. The free energy values are reported in kcal mol−1. The landscape is obtained by summing over all the microstates of the 2,000 state MSM fromi=1 toNusing the following equationwhereπiis the probability of stateiin the MSM, andhi(x,y) is the normalized histogram of the variablesxandyrestricted to the MSM statei. Figure 2: Conformational landscape of c-src tyrosine kinase. The conformational landscape generated using r.m.s.d. of A-loop residues (404–424) and difference of the distance between Glu310-Arg409 and Lys295-Glu310 residue pairs as the order parameters reveals multiple intermediates along the activation pathway. The free energy values are reported in kcal mol −1 . The landscape is obtained by summing over all the microstates of the 2,000 state MSM from i =1 to N using the following equation where π i is the probability of state i in the MSM, and h i ( x , y ) is the normalized histogram of the variables x and y restricted to the MSM state i . 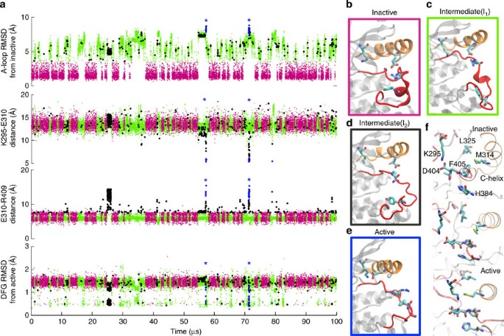Figure 3: Kinetics of the c-src kinase activation. MSM of the kinase conformational change reveals novel intermediate states along the activation pathway and provide a measure of the activation/deactivation timescales. (a) Variation of key structural metrics as a function of time along the activation trajectory obtained using the MSM. MSM trajectories are calculated using a kinetic Monte Carlo algorithm to generate a trajectory of (τ=5 ns) microstate jumps, and selecting at random (uniformly) a simulation snapshot to report observables at each time step. The r.m.s.d. of the activation loop is calculated using heavy atoms of residues 404–424. The following atoms were used for the calculations of distances between residues: Lys295(NZ atom in thegroup), Glu310 (CD atom in the COO−group) and Arg409 (CZ atom in the guanidinium group). Different colours represent the different conformational states of the c-src kinase. Inactive (b), intermediate states I1(c), I2(d) and active (e) states are shown in magenta, green, black and blue, respectively, with active state also marked with an asterisk. (f) These four conformational states could be further subdivided into states with different conformations of DFG-motif and R-spine. Full size image Figure 3: Kinetics of the c-src kinase activation. MSM of the kinase conformational change reveals novel intermediate states along the activation pathway and provide a measure of the activation/deactivation timescales. ( a ) Variation of key structural metrics as a function of time along the activation trajectory obtained using the MSM. MSM trajectories are calculated using a kinetic Monte Carlo algorithm to generate a trajectory of ( τ =5 ns) microstate jumps, and selecting at random (uniformly) a simulation snapshot to report observables at each time step. The r.m.s.d. of the activation loop is calculated using heavy atoms of residues 404–424. The following atoms were used for the calculations of distances between residues: Lys295(NZ atom in the group), Glu310 (CD atom in the COO − group) and Arg409 (CZ atom in the guanidinium group). Different colours represent the different conformational states of the c-src kinase. Inactive ( b ), intermediate states I 1 ( c ), I 2 ( d ) and active ( e ) states are shown in magenta, green, black and blue, respectively, with active state also marked with an asterisk. ( f ) These four conformational states could be further subdivided into states with different conformations of DFG-motif and R-spine. Full size image These results suggest that the A-loop has to unfold before the conformational changes in the C-helix. This observation is broadly consistent with previous computational studies related to not only Src family tyrosine kinases [17] , [18] , [23] , [24] , [25] , [27] but also serine-threonine kinases [22] . In particular, the Src kinase conformational landscape obtained from independent umbrella sampling simulations by Meng and Roux [27] also reveals similar intermediate states. In the current study, extensive sampling of possible catalytic domain conformations is obtained, whereas Meng and Roux [27] have reported conformational landscape with the A-loop in only open conformation. To present a direct comparison between these studies, we have now reported a conformational landscape obtained using MSM and umbrella sampling results [27] including all conformations of A-loop ( Supplementary Fig. 3 ). The computed population of active (unphosphorylated active-like) conformation from the umbrella sampling calculations reported by Meng and Roux [27] was found to be 0.002, which is in agreement with the value of 0.0018 obtained in this study. Similarly, a previous computational study of Hck kinase (a member of the Src family of tyrosine kinases with high structural similarity to c-src) also reported the existence of two intermediate states along the pathway between the inactive and active state kinase [18] . However, there are noteworthy differences with the intermediate states reported in the present study that could be potentially exploited for drug design purposes. The intermediate (I 1 ) of Hck involves partial unfolding of A-loop and has an intact Glu310-Arg409 ion pair, which is similar to the Intermediate I 1 of c-src (the difference lies in the extent of unfolding of A-loop). However, the second intermediate of Hck is distinct from the intermediate I 2 of c-src. The A-loop in Hck intermediate I 2 is not fully unfolded, whereas it is completely unfolded in c-src. The Lys295-Glu310 ion pair is not formed in c-src, whereas it is formed in the Hck kinase. The binding of 8-anilino-1-napthalene sulphonate (ANS) to the allosteric site in c-src requires complete unfolding of A-loop. Furthermore, Glu310-Arg409 ion pair stabilizes the partially unfolded states of A-loop, with the DFG-motif end of the A-loop in its inactive conformation. Therefore, ANS can only bind to intermediate I 2 of c-src with broken Glu310-Arg409 ion pair. Therefore, intermediate states of Hck kinase would not be able to bind ANS molecule because both these intermediate states have partially unfolded A-loop. Furthermore, intermediate I 2 of Hck kinase has partially formed Lys295-Glu310 ion pair that blocks the primary ANS-binding site. These observations and the simulation results show that the methods outlined in this study could be used for successfully identifying the subtle structural differences between the kinases with high structural and sequence similarity. Recent computational studies on epidermal growth factor receptor kinase have revealed a partially unfolded conformation of C-helix. Our results indicate that for the Src kinase, the C-helix remains folded during activation as indicated by the high helical content and stable solvent accessible surface area of the C-helix ( Supplementary Fig. 4 ). This observation is consistent with the H-D exchange experiments and bioinformatic analysis of the intrinsic disorder at the C-helix in Src kinase [37] . Diversity within intermediate states of c-src The conformational landscapes also show a rich diversity within the intermediate states because of the partially unfolded states of A-loop and the multiple conformational states of DFG-motif (Asp404-Gly406) and R-spine(Leu325, Met314, Phe405 and His384; Supplementary Figs 5–8 ). DFG residues (Asp404, F405 and G406) at the N-terminal end of the A-loop play a critical role in activation of kinases. The crystal structures of active and inactive states of c-src have the DFG motif in the ‘DFG-in’ states [29] , [30] . The DFG-out state is not accessible in the conformational landscape of ATP-bound c-src ( Supplementary Fig. 8 ) owing to the interaction between the DFG-aspartate residue and the Mg 2+ ions bound to the phosphate groups of ATP and steric clash between DFG-phenylalanine and the ATP in the DFG-out state. The DFG motif does not completely flip in the simulations but it still shows considerable fluctuations along the activation pathways. The variation of root mean squared deviation (r.m.s.d.) of the DFG motif (from the active state) with respect to the r.m.s.d. of the A-loop (from the inactive state) shows that DFG motif adopts multiple intermediate conformations because of the movement of the individual loop residues during activation ( Supplementary Fig. 6 ). In the active ‘DFG-in’ state, F405 participates in the formation of the R-spine, which is the hallmark of the active c-src. For the formation of R-spine, F405 has to flip partially to make space for the M314 (in the C-helix) to occupy the gap between L325 and F405 ( Fig. 3f ). The fluctuations of the positions of these individual residues also show that a rich diversity of conformations exists within individual metastable basins corresponding to active, inactive and intermediate states. Deactivation timescales are faster than activation timescales The first eigenvector of the transition probability matrix T ij (includes transition probabilities from state i to state j ) provides the estimate of the equilibrium population of all states in MSM. The equilibrium probabilities estimated from the microstate MSM with respect to the r.m.s.d. of the state from the inactive and active states show that the inactive state is the most populated state ( P inactive ~0.56) and the active state is one of the least populated states ( P active ~0.001; Supplementary Fig. 9 ). These observations are consistent with a free energy barrier of 3.8 kcal mol −1 between the inactive and active states. These values also suggest that the active state is visited transiently in the conformational landscape and requires either binding of a substrate or phosphorylation of Tyr416 to remain in the active state [11] . The A-loop remains extended in the intermediate and active states, thereby increasing the possibility of stimulatory transphosphorylation of Tyr416. The slowest process occurring on the conformational landscape of c-src involves population flow from inactive state to a partially active state with A-loop fully unfolded and R-spine partially aligned. ( Supplementary Fig. 10 ) Furthermore, the Glu310-Arg409 were hydrogen bonded in the partially active state indicating that the slowest dynamical process involves transition between the inactive state and a microstate with a fully unfolded A-loop. Figure 3a shows a 100-μs trajectory generated from the MSM using kinetic Monte Carlo scheme starting from the inactive state. Two activation events are observed in this trajectory as denoted by an asterisk. Colours of the dots indicate the four macrostates (active, inactive, I 1 and I 2 ) as shown in Fig. 3b–e . The mean first passage time (MFPT) for activation (defined as transition between states with r.m.s.d. closest to the inactive and active state crystal structures) is calculated to be ~106 μs, whereas the MFPT for deactivation is found to be ~21 μs. Such long timescales extracted from MSM analysis may appear inconsistent with the relatively small free energy barriers between the inactive, active and intermediate states observed in the potential of mean force (PMF) plot shown in Fig. 2 . However, it is worth pointing out that absolute transition rates in complex multidimensional systems depend on a multiple structural and dynamical factors that may remain hidden in a PMF projection onto a subspace of a few order parameters. Other projections for the 100-μs trajectory are shown in Supplementary Fig. 11 . The R-spine alignment is coupled to the C-helix rotation and displacement but the couplings are loose. The R-spine fluctuates between active, inactive and intermediate conformations ( Fig. 3f ) regardless of the conformation of the catalytic domain. R-spine alignment takes place more frequently in the intermediate states indicating that partial unfolding of the A-loop facilitates the rotation of the C-helix. Our results indicate that, although there is one broad pathway connecting the active and inactive states but if the fluctuations in individual residues comprising ‘DFG’-motif and R-spine are considered, it leads to an ensemble of activation pathways with comparable flux, which provides a more fine-grained view of the kinase activation ( Supplementary Fig. 12 ). Relating fast activation to slow rate of autophosphorylation The experimentally observed timescale for Src-family tyrosine kinase autosphosphrylation at residue Tyr416 is on the order of minutes [38] , whereas the timescale of the conformational transitions associated with kinase activation obtained from the present computational analysis is 110 μs. To relate these vastly disparate timescales, we constructed a kinetic model describing the time evolution of activated kinase population using the thermodynamic and kinetic data extracted from the atomistic simulations following the reaction scheme included below. where I is the inactivated state, A is the unphosphorylated active state, A* is phosphorylated (locked) active state, k IA is the activation rate and k AI is the deactivation rate. The rate k trans−p is the rate of kinase phosphorylation, which requires intermolecular encounter with another active kinase (see Methods for model description). A key result from the present analysis is that the catalytic domain undergoes fast exchange between the inactive state and an active-unphosphorylated conformation. Because of the low bimolecular encounter frequency with catalytically active kinases, the fast exchange effectively leads to kinase populations that are in pseudo equilibrium. Time evolution of active phosphorylated kinase population shows a lag or induction time, which is an experimentally observed feature ( Supplementary Fig. 13a ) [38] , [39] . The lag time indicates the slow initial build up of active kinases. As some kinases reach active state by fluctuations, they become available to seed and initiate the autophosphorylation of other kinases, which then leads to a sharp increase in active kinase population. The model also correctly predicts the experimentally observed relationship between time evolution of active kinase population and enzyme concentration, rates of autophosphorylation and activation. Our model results predict that the time evolution of active kinase population is sensitive to changes in the effective equilibrium constant ( K eq ) between inactive and active-unphosphorylated states ( Supplementary Fig. 13 ). The typical experimental values of t 1/2 (time taken for half the kinases to be in active state) is in minutes. Under conditions that are representative of experiments, the limits on K eq values consistent with the range of experimental t 1/2 values can be estimated using the model. Assuming the rate of autophosphorylation to be 10 μM −1 s −1 , total enzyme concentration [ C tot ]=1 μM and the value of K eq =740 calculated from the MSM equilibrium populations, the t 1/2 values is found to be 8.2 min, which lies in the experimental observed range of 5< t 1/2 <10 min (Moarefi et al. [38] ). Keeping c-src inactive by stabilizing intermediate states Mechanistic understanding of the kinase activation process could be harnessed for the design of novel inhibitors. In this study, we have predicted the existence of metastable intermediate states I 1 and I 2 , which could be stabilized to block the activation process. Coincidently, a recent crystal structure of cyclin-dependent kinase 2 (CDK2; from the CMGC family of the serine/threonine kinases) bound to ANS has structural features similar to the intermediate I 2 of c-src ( Supplementary Fig. 14 ) [40] . Furthermore, ANS molecules were bound to the pocket between the C-helix and β 4 , which is different from typical kinase inhibitors that bind to the ATP-binding pocket or the adjacent hydrophobic pocket ( Supplementary Fig. 15 ) [41] . From the activation mechanism of c-src kinase, it is evident that the binding of any drug in the region between C-helix and the β-sheets in the N-terminal lobe would block the displacement and/or rotation of the C-helix, thereby trapping the kinase in a partially active intermediate state. Simulations of ANS-bound intermediate I 2 from c-src were performed to assess the interactions of the drug molecule with the c-src residues and to ascertain structural changes induced by the drug binding. The structures obtained from the simulations of ANS-bound c-src reveal outward movement of the C-helix as compared with the ATP-bound c-src, which is significantly different from both the active and inactive crystal structures of c-src ( Fig. 4 ). The displacement of the C-helix would not only block the activation of the kinase but also interfere with the binding of the substrate. The R-spine alignment is also disrupted owing to ANS binding, indicating that the ANS also interferes with the rotation of the C-helix, which could potentially suppress the catalytic activity of the kinase ( Supplementary Fig. 16 ). The simulations also show that ANS molecule sits directly between the Lys295 and Glu310 residues, thereby blocking any possibility of hydrogen bond formation between these residues, which is essential for the inward movement of C-helix ( Supplementary Fig. 17 ). Furthermore, strong hydrogen bond formation is observed between the sulphonate group of ANS and Lys295 ( Fig. 4 ). The primary ANS-binding pocket is hydrophobic in nature that interacts favourably with the naphthalene and the phenyl rings in the ANS molecules ( Supplementary Fig. 18 ). The phenyl ring was found to interact with Phe278, Phe307 and Leu297 residues, whereas the naphthalene ring interacts with Phe405, Ala403, Val323, Leu325 and Ile336 residues. 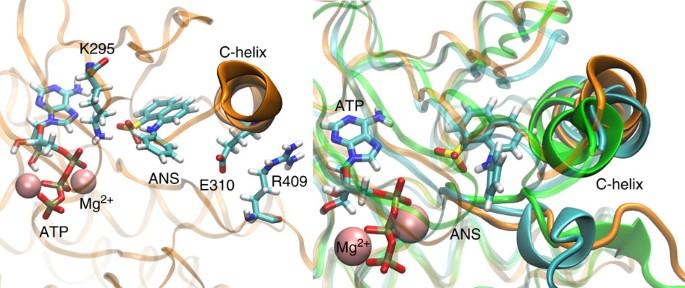Figure 4: Mechanism of ANS-induced stabilization of intermediate I2. (Left) ANS binding to the allosteric site adjacent to C-helix in c-src kinase stabilizes the intermediate conformation by blocking the interactions between Lys295 and Glu310. The hydrogen bond formation between Lys295 and Glu310 is required for the locking of the C-helix in the active conformation. The sulphonate group in the ANS forms a hydrogen bond with the Lys295, thereby locking it in its inactive conformation. (Right) ANS binding also pushes the C-helix away from the ATP-binding pocket. Superimposition of the crystal structures of the inactive (cyan) and active (green) states of ATP-bound c-src kinase with the ANS-bound src-kinase (orange) reveals the distinct conformation of the C-helix in presence of ANS. Figure 4: Mechanism of ANS-induced stabilization of intermediate I 2 . (Left) ANS binding to the allosteric site adjacent to C-helix in c-src kinase stabilizes the intermediate conformation by blocking the interactions between Lys295 and Glu310. The hydrogen bond formation between Lys295 and Glu310 is required for the locking of the C-helix in the active conformation. The sulphonate group in the ANS forms a hydrogen bond with the Lys295, thereby locking it in its inactive conformation. (Right) ANS binding also pushes the C-helix away from the ATP-binding pocket. Superimposition of the crystal structures of the inactive (cyan) and active (green) states of ATP-bound c-src kinase with the ANS-bound src-kinase (orange) reveals the distinct conformation of the C-helix in presence of ANS. Full size image Long range dynamic coupling between residues in c-src Allosteric communication lies at the heart of the kinase activation process with long-range inter and intradomain communication networks controlling the conformation of the enzyme [42] . Mutual information analysis that provides a measure of long-range coupling between residues by calculating the correlation between the motions of their backbone and side-chain torsion angles is used to identify allosteric couplings in c-src kinase [43] . Variation of mutual information as a function of C α atom distance between residue pairs shows that there is significant correlation between residue pairs even 20 Å apart from each other ( Supplementary Fig. 19 ). The long-range coupling between residues is also evident from the mutual information values between each residue pair in c-src kinase ( Fig. 5 ). Furthermore, a visual inspection of the matrix also shows the presence of strong local coupling in different regions of kinase ( Supplementary Fig. 20 ). For example, activation segment (residues 404–432) not only shows long-range coupling, but it also forms a strong local network of coupled residues indicating a cooperative unfolding during activation. The second locally coupled network of residues comprises the loop at the C-terminal end of αE, which forms a β-sheet with the unfolded A-loop in the active state. Mutual information values for the key residues in catalytic domain show that all the residues in electrostatic network, R-spine and DFG motif are strongly coupled with the A-loop ( Supplementary Figs 21,22 ). Furthermore, residues F405 (DFG motif), Glu310, Arg409 and Tyr416 also show a strong coupling with C-terminal lobe residues. Such strong coupling not only offers an avenue for targeted drug design but also explains the origin of the molecular resistance and the deleterious effects of large number of point mutations in the catalytic domain on the kinase activity. 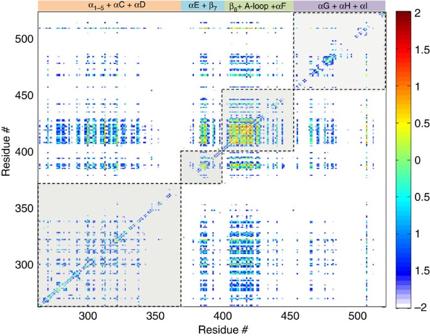Figure 5: Mutual information between residues in c-src kinase. Hierarchical clustering of significant mutual information values identifies four regions (shown as squares) within the catalytic domain, which have significant dynamical correlation between them. The most strongly coupled cluster involves the residues in the A-loop region that cooperatively unfold during the activation process. Colours indicate the log of the mutual information value. Figure 5: Mutual information between residues in c-src kinase. Hierarchical clustering of significant mutual information values identifies four regions (shown as squares) within the catalytic domain, which have significant dynamical correlation between them. The most strongly coupled cluster involves the residues in the A-loop region that cooperatively unfold during the activation process. Colours indicate the log of the mutual information value. Full size image The A-loop region is also coupled to myristate-binding pocket region in c-src at the base of the C-terminal lobe. Myristoylation has been shown to regulate c-src activity and stability [44] but there are no crystal structures of the myristoylated c-src. It has been shown via NMR experiments that myristate can bind to a pocket in c-src, which is similar to the myristate-binding pocket in c-Abl (a tyrosine kinase with similar fold as c-src) [29] . Drugs targeting the myristol-binding pocket have been shown to allosterically modulate the conformation of A-loop and ATP-binding pocket in c-Abl kinase [3] . Our results indicate that drugs targeting the myristate-binding pocket in c-src could also serve as allosteric modulators of c-src kinase activity. In this study, we have used a combination of pathway generation technique (string method in collective variables [45] , [46] ) and massive distributed computing coupled with MSMs for studying long timescale phenomena [47] . We showed that this method can efficiently capture kinetics with short independent trajectories several orders of magnitude shorter than the timescale of the process under investigation. This method also represents a much more efficient use of simulation time than simply running a long brute force simulation of the same length. For example, to observe 10 activation events of c-src kinase in a single trajectory, a total simulation time of ~1,100 μs would be required. Here we obtained converged timescales and conformational landscapes in ~100 μs starting from a conformational transition pathway determined via the string method. Our results also show that network models of conformational change present a more natural framework for describing enzyme dynamics on a complex conformational landscape as compared with a linear reaction coordinate analysis or few state models. MSMs are well developed for studying global conformational rearrangements such as protein folding [35] , but these models have not been used extensively for studying conformational changes in enzymes. This study represents one of the fist application of novel MSM approaches for studying complex conformational changes in enzymes and provides pointers for further methodological advances in this direction. Long timescale simulation of c-src kinase reported in this study has provided novel insights into the mechanism of kinase activation. However, there are several caveats worth noting. First, we have not performed the simulations of the catalytic domain along with its two regulatory domains, which must presumably influence the kinetics of activation. Second, it is likely that the activation mechanism is also dependent on the phosphorylation state of Tyr416. This study provides an extensive database of possible conformations of the catalytic domain, which can be used as a set of templates for obtaining starting configurations for simulations of catalytic domain with phosphorylated Tyr416 and catalytic domain with bound regulatory domains. Owing to these extensive set of distinct starting configurations, their conformational landscapes could be quickly sampled in parallel. Simple model of kinase autophosphorylation predicts the presence of induction time in the time evolution of active kinase population. According to the activation timescales reported in this study, the rate of autophosphorylation is the limiting step in the kinase phosphorylation process. However, the time evolution of active kinase population was found to be sensitive to the equilibrium constant ( K eq ) relating inactive to active (unphosphorylated) state equilibrium populations. For Src family kinases in the downregulated state (both regulatory domains bound to the catalytic domain and C-terminal Tyr527 phosphorylated), it has been observed that induction time increases significantly as compared with the kinase with unphosphorylated Tyr527 (Moarefi et al. [38] ). Our results suggest that shift in the equilibrium population of active (unphosphorylated) kinases from 10 −3 to 10 −4 would change the induction time from several minutes to hours. These results support the view that fast kinase conformational fluctuations at the 10–100-μs timescale control the observed macro timescale behaviour. We also predict the existence of binding pocket for novel allosteric inhibitors, the ANS-binding pocket adjacent to C-helix in c-src. On the basis of the binding interactions of ANS with c-src, novel allosteric inhibitors that span the ATP-binding pocket and the ANS-binding site or inhibitors that span both the ANS sites could be designed [41] . This fragment-based inhibitor design approach has been used to design CDK2 inhibitor AT7519, which consists of two covalently linked fragments that bind to different regions of the targeted kinase [48] , [49] , [50] . Allosteric inhibitors targeting this site would not only help in selective inhibition of kinases but would also be useful for understanding the function of a single kinase in a complex cellular signalling milieu [51] . The present results provide a description of the thermodynamic and kinetic factors underlying the activation of c-src kinase with unprecedented atomistic detail. Src-family kinases share a conserved protein fold and are highly homologous in sequence. This raises a host of fascinating questions about the similarities of their activation mechanisms. If there are subtle differences in their activation mechanisms (which could be studied using the methodologies used in this study), then these differences could be harnessed for future design of selective inhibitors for individual members of Src family. Generation of initial pathway using string method The inactive (PDB ID: 2SRC) [30] and active (PDB ID: 1Y57) [29] X-ray structures of human c-src kinase were used as the two end point conformations for the generation of the MFEP. Only the catalytic domain residues (W260–T521) are included in the simulation set-up. The initial pathway used in adaptive sampling simulation described below was generated by a two-steps procedure to filter out the noise in pathways computed using the string method in high-dimensional spaces in the space of collective variables [45] , [46] . The methodology combines principal component analysis to identify a number of relevant modes that can effectively describe the transition with a smoothing procedure of a representative path from the ensemble of projected ones. Principal component analysis was performed on an ensemble of 30 paths that corresponded to iteration 71–100 of the inactive-to-active human c-src tyrosine kinase conformational transition that was obtained in Gan et al. [24] Fifteen principal components were identified such that the difference with the original ones is less than the difference between the projected pairs of paths. The average of the 30 projected paths was taken and a smoothing algorithm was applied. The strategy we employ to smoothen a string defined in a high-dimensional space is to minimize the following objective function: where t i is the unit tangent vector between a pair of images along the string and R i is the distance of image i from all the replicas of the same image in the ensemble of paths. k a and k d are scalar parameters to be chosen by the user that describe the weight of different terms and are equal to 1.0 and 0.03, respectively, while δ is a threshold value. One thousand steps of steepest decent minimization were performed. The final path was then transformed back to original Cartesian coordinate system and was used to initiate the adaptive sampling process [52] on Folding@home. Starting conformations for the simulations were taken from the 51 snapshots along the smoothed MFEP. Simulation details Distributed MD simulations were performed using GROMACS [53] on the Folding@home [28] computing platform. The CHARMM22 (Brooks et al. [54] ) force field was used for protein and ligands along with TIP3P [55] water model. The all-atom structures were then solvated in a truncated octahedral solvent box constructed from a 80 × 80 × 80 Å 3 cube with TIP3P water molecules such that water extended at least 10 Å away from the surface of the protein; 22 Na + ions and 19 Cl − ions were added to the system to neutralize the charge, corresponding to a salt concentration of ~150 mM. Covalent bonds involving hydrogen atoms were constrained with LINCS [56] and particle mesh Ewald [57] was used to treat long-range electrostatic interactions. The structures obtained after an initial equilibration for 1 ns at constant temperature and pressure and with constraints on the heavy atom positions were used as the starting conformation for the distributed MD simulations. Production MD simulations were carried out at constant temperature and pressure of 300 K and 1 atm, respectively, with a time step of 2 fs. Two sets of simulations were started using the initial structures generated using the protocol described above. The first set of ~12,000 simulations were started from the 51 snapshots along the string method pathway for an aggregate simulation time of 150 μs on the Folding@home platform. To ensure that the simulations started from the string method do not give a biased conformational landscape, another set of 12,000 simulations were performed starting from only the active and inactive states of c-src kinase. The aggregate simulation time of 350 μs was obtained for this set using the Folding@home platform. The conformational landscapes obtained using the second data set do not reveal new regions of landscape as compared with the conformational landscape obtained using the 150-μs simulations performed using the snapshots from the string method pathway. Simulations of c-src kinase catalytic domain were also performed in the AMBER99sb-ildn force field ( total duration ~50 μs) to test the dependence of the simulation results on the choice of force field. These simulations were started from the MSM states obtained from the simulations of kinase catalytic domain in CHARMM22 force field. The simulations were found to be independent of the choice of force field. Adaptive sampling algorithms based on MSMs [52] , [58] were used to efficiently sample the conformational landscape of c-src tyrosine kinase. The initial structures for adaptive sampling rounds were chosen from the MSM states with the minimum population. In all, we performed two rounds of adaptive sampling and a total of 24,000 simulations with a total duration of 500 μs. Trajectory snapshots were recorded every 100 ps. The distribution of total number of simulations versus the simulation length is shown in Supplementary Fig. 23 . Simulations of c-src intermediate with ANS molecules bound to the allosteric site adjacent to the C-helix were performed to assess the ability of ANS to block activation of c-src tyrosine kinase. Two sets of simulations were performed: first, with one molecules of ANS bound to the protein and, the second, with two molecules of ANS bound to the protein. The crystal structure of CDK2 in complex with two molecules of ANS (PDB ID: 3PXF) [40] was used as a template to align the residues of the c-src intermediate within 5.0 Å of the ANS-binding pocket. The force filed parameters for ANS were obtained using GAFF [59] . The aligned kinase structure along with the ANS molecules was then solvated in a truncated octahedral solvent box with TIP3P water molecules and ions added to neutralize the charge, corresponding to a salt concentration of ~150 mM. The corresponding systems were minimized using GROMACS for 100,000 steps and then equilibriated for 2 ns at constant temperature and pressure of 300 K and 1 atm, respectively. A total of 2000 distributed MD simulations were started from the two structures for an aggregate simulation time of 50 microseconds using the simulation protocols outlined above. Markov state models Our methods draw on kinetic network models called Markov state models (MSMs) that are built from extensive molecular dynamics simulations using Folding@home [28] distributed computing architecture to describe a protein-intrinsic dynamics. Similar to a map of a molecule’s free energy landscape, an MSM provides a reduced view of the ensemble of spontaneous fluctuations the molecule undergoes at equilibrium. These models provide the population and transition rates between key conformational states of protein [31] , [32] , [36] . The MSMBuilder [60] software was used to build MSMs of the conformational landscape of c-src tyrosine kinase. Conformations were clustered using a subset of heavy atoms identified using the root mean square fluctuations of atoms after subtracting the inactive-state root mean square fluctuation values. The subset of atoms include all heavy atoms from the N-terminal lobe residues 270–340, and A-loop residues 404–424 were used for the clustering and construction of the MSM ( Supplementary Fig. 24 ). MSMs describe the conformational dynamics of proteins in terms of jumps between the microstates obtained from the clustering of the simulation data set into discrete states. The transition probability matrix T ( τ ) includes the probability of transitions from state i to state j in a certain time interval τ and are estimated by counting the number of transitions n ij observed between time t and t + τ , and normalizing n ij with the sum of all transitions from state i . To enforce detailed balance(which ensures that population of states is conserved), a maximum likelihood estimate of the transition probability matrix that follows the detailed balance is obtained. The transition probability matrix can be used to obtain the population of the system at any time using the following relationship: where p ( t ) is the vector of state population at time t . The eigenvalue/eigenvectors spectrum of the transition matrix gives information about the aggregate transitions between subsets of states in the model and what timescales these transitions occur on [61] . The equilibrium population of the individual states are estimated from the first eigenvector of the transition probability matrix. The timescales of the dynamical processes occurring on the conformational landscape of c-src can be obtained by estimating the eigenvalues of this matrix. The eigenvalues μ of the transition probability matrix are related to the implied timescales 1/ k of transitions via the following expression: The 2000-state model decomposition yielded a good balance between state connectivity and adequate transition sampling. The model also provided converged implied timescales as a function of lag time, which is used as a measure of the Markov nature of the model ( Supplementary Fig. 1 ). A lag time of τ =5 ns was determined to be suitable by building a series of MSMs at different lag times to find a region where the spectrum of implied timescales are relatively insensitive to lag time. Transition Path theory was used to analyse the distribution of activation pathway fluxes from inactive to active states. Committor values and MFPTs were computed for each state using methods described in the literature [62] , [63] , [64] . Similar simulation and analysis protocol has been successfully used earlier for the study of Hck kinase [18] , where initial structures of the catalytic domain were taken from the pathway generated using targeted MD simulations. Short simulations (total simulation time of 1 μs) from these initial structures were performed and subsequently analysed using kinetic network models for studying the conformational transition between active and inactive state. Mutual information The excess mutual information was computed for all protein torsion angles (backbone dihedrals φ , ψ and side chain χ angles (only the first χ angle for proline)) throughout the simulations to capture nonlinear correlated motions of residues in an unbiased, statistically robust manner. The following formula was used for the calculation of mutual information between residue pairs [43] : The average of the mutual information computed from 10 iterations of scrambled data was subtracted from the mutual information values computed from the simulation data to filter out correlations that are not statistically significant. Model for transautophosphorylation of kinases Residue Tyr416 in c-src kinase is phosphorylated to lock the kinase in the active conformation, thereby enhancing its ability to catalyse the phosphate transfer from ATP to the substrate. The thermodynamic and kinetic data reported in this study are used to build a kinetic model of kinase autophosphorylation following the reaction scheme included below. where I is the inactivated state, A is the unphosphorylated active state, A* is phosphorylated (locked) active state, k IA is the activation rate and k AI is the deactivation rate. The rate k trans−p is the rate of kinase phosphorylation, which requires intermolecular encounter with another active kinase. The time evolution of different state of kinase in the solution can be described using the following ordinary differential equations. The rate of phosphorylation is much slower than the activation/deactivation rates because it involved a diffusion-limited bimolecular encounter between two active kinases. The kinase activation timescales measured in this study are of the order of 100 μs. The set of equations (7)–(9), could be simplified by assuming a pseudo equilibrium between inactive and unphosphorylated active state. The inactive ( P I ) and unphosphorylated active state ( P A ) equilibrium populations obtained from the MSMs results reported in this study are used for estimating K eq . The pseudo equilibrium assumption is valid under the following condition: The total concentration of protein [ C I ]+[ C A ]+[ C A* ]=[ C tot ] is fixed, which provides the following relationship between [ C A ] and [ C A* ]. The equation (9) is simplified to the following ordinary differential equation by substituting [ C A ] expression from the equation (15). This initial value problem can be solved numerically or analytically using P A* t =0 =0 and [ C tot ]=1 μM as the initial conditions. The analytical solution of the above initial value problem has the following form: Substituting the values t = t 1/2 , P A* =0.5 in the above equation provides the expression for the time required for half the kinases to be phosphorylated. This expression is used to obtain limits on the value of K eq by comparing the experimental t 1/2 values with the model predictions for different values of K eq . For k trans−p =10 μM −1 s −1 , [ C tot ]=1 μM and 1 min < t 1/2 <10 min, the K eq values lie in the range (130,880). The value of K eq calculated from the MSM equilibrium populations is 740. Similarly, for the predicted value of K eq , the limits on k trans−p [ C tot ] were found to be (8,80) s −1 . ADP release has been identified as the slowest step in the kinase catalytic cycle for a variety of kinases [65] . In the model above, the effect of slow ADP release process could be captured by decreasing the autocatalytic effect of the active phosphorylated kinase population. The ADP-bound active state cannot phosphorylate other active kinases and has to release ADP and bind to ATP to catalyse the next phosphate transfer reaction. This effect can be captured by lowering the value of the rate of autophoshorylation k trans−p . The value of k trans−p was chosen to be 10 μM −1 s −1 owing to the rate-limiting effect of ADP release. The value of k trans−p =10 μM −1 s −1 at the total kinase concentration of 1 μM translates to an effective phosphorylation rate of 10 s −1 . The experimental ADP release rate lies in the range (1,100) s −1 (Adams et al. [65] ). Therefore, the results from the simplified model proposed above are not expected to change significantly because of incorporation of the ADP release in the model. However, we have also included details of the kinetic model with ADP release in the Supplementary Methods to substantiate this claim. Procedure for generating MSM trajectories Several simulation studies have reported methodologies for obtaining kinetics from network model [66] , [67] , [68] . The time course of observables were obtained by using a kinetic Monte Carlo scheme on the transition probability matrix T , where T ij represent the probability of transition from state i to j . For a MSM trajectory in state i at time t , the next state visited at time t + τ is estimated using the following scheme: 1 Generate a random number lying between [0,1]. 2 Calculate the probability R ik for all states given by R i , k =Σ j =1 k T ij . 3 If the generated random number lies between R i , k and R i , k +1 , then the state k is chosen for transition. 4 Select a random snapshot from the conformations assigned to state k . All conformations assigned to a particular microstate are structurally similar (because of the small size of the microstate) and they interconvert at a timescale smaller than the lag time. Therefore, the representative conformation for state k is chosen randomly (uniformly) from all the conformations assigned to this state. 5 Calculate the observables from the selected conformation. Procedure for calculating MFPTs between states from MSMs Singhal et al. [69] , [70] have reported a detailed procedure for the calculation of MFPT from MSMs. In brief, MFPTs are calculated from a set of linear equations that are based on the MSM transition probability matrix. MFPT is defined as the average time taken to get from a particular state i to a any state j in the final (in this case all active or inactive states) set of states. The MFPT can be defined conditionally based on the following expression: where the sum is over all transitions from i to j . The MFPT( i ) is the sum of the time it takes to transition from state k to i and MFPT( k ), which gives where sum is over all the edges leading from state i . Similar equations can be written for MFPT from all states to state j to generate a system of linear equations, which can be solved for MFPT( i ). How to cite this article: Shukla, D. et al. Activation pathway of Src kinase reveals intermediate states as targets for drug design. Nat. Commun. 5:3397 doi: 10.1038/ncomms4397 (2014).